Granulocyte macrophage colony-stimulating factor is required for aortic dissection/intramural haematoma Aortic dissection and intramural haematoma comprise an aortopathy involving separation of the aortic wall. Underlying mechanisms of the condition remain unclear. Here we show that granulocyte macrophage colony-stimulating factor (GM-CSF) is a triggering molecule for this condition. Transcription factor Krüppel-like factor 6 (KLF6)-myeloid-specific conditional deficient mice exhibit this aortic phenotype when subjected to aortic inflammation. Mechanistically, KLF6 downregulates expression and secretion of GM-CSF. Administration of neutralizing antibody against GM-CSF prevents the condition in these mice. Conversely, administration of GM-CSF in combination with aortic inflammation to wild-type mice is sufficient to induce the phenotype, suggesting the general nature of effects. Moreover, patients with this condition show highly increased circulating levels of GM-CSF, which is also locally expressed in the dissected aorta. GM-CSF is therefore a key regulatory molecule causative of this aortopathy, and modulation of this cytokine might be an exploitable treatment strategy for the condition. Aortic dissection and intramural haematoma comprise a potentially life-threatening aortopathy involving separation of the aortic wall [1] , [2] , [3] , [4] , [5] , [6] . The two conditions are distinguished by a tear in the aortic intima as present in the former classical form of aortic dissection, which results in blood flow into the aortic wall and is absent in the latter form of intramural haematoma with bleeding confined within the aortic wall. This aortopathy is presently understood to be a continuum, with the latter a variant and precursory condition of the former [7] , [8] , [9] . Advancements in the understanding of genetic underpinnings (for example, ACTA2 ) [10] , [11] , clinical/epidemiological aspects (for example, The International Registry of Acute Aortic Dissections (IRAD)) [4] , [5] as well as biochemical approaches (for example, smooth muscle biomarkers) [5] , [6] have been made in the last decade, but underlying mechanisms have remained obscure owing much to lack of a reliable animal model. Recent advancements in understanding mechanisms of aortic disease have stemmed from hallmark studies in the genetically fragile Marfan aorta, which have shown that transforming growth factor β (TGFβ) and its downstream intracellular kinase signalling pathways play a central role in the pathogenesis [12] , [13] , [14] . In contrast, an inflammatory pathway is thought to be a major component of aortic conditions in the atherosclerotic/degenerative aorta seen in the typical elderly patient [15] , [16] . Commonalities and differences in mechanisms as well as relative contributions of underlying processes in these different aortic conditions have only begun to be unravelled. In the present study, we sought to address the underlying mechanisms of aortic dissection/intramural haematoma, and to understand the triggering mechanism of the condition. Krüppel-like factor 6 (KLF6) is a transcription factor that has been shown to be robustly expressed in macrophages [17] , and to regulate inflammatory fibrotic diseases of multiple organs including the liver [18] and kidney [19] . In the present study, we hypothesized that this factor might regulate pathogenic mechanisms underlying aortic disease, and observed that mice deficient for KLF6 in macrophages when subjected to aortic inflammation manifest aortic dissection/intramural haematoma. Intriguingly, we find that the inflammatory cytokine, granulocyte macrophage colony-stimulating factor (GM-CSF) [20] , plays a central role in onset of this condition. Administration of neutralizing antibody against GM-CSF prevents the condition in these mice. Conversely, administration of the cytokine in combination with aortic inflammation to wild-type mice is sufficient to induce the condition, suggesting general effects. Clinically, patients with aortic dissection show elevated circulating levels of the cytokine, which is also expressed in the dissected aorta. GM-CSF is therefore a key regulatory molecule causative of aortic dissection/intramural haematoma. Aortic aneurysm with inflammation in Klf6 heterozygous mice We initially found that mice heterozygously depleted for Klf6 manifest a phenotype of exacerbated aortic aneurysm (defined as greater than 50% increase in the external aortic diameter with a conserved aortic wall) [21] , [22] , when subjected to aortic inflammation (2 weeks infusion of angiotensin II (AngII) with local application of calcium chloride (CaCl 2 )). Histological findings showed enlargement of the aortic lumen with a fragile aortic wall and further fibrotic tissue deposition compounded with marked infiltration of macrophages (Mac3-positive cells) ( Fig. 1a–e ). Mechanistically, increased expression of matrix metalloprotease-9 ( MMP9 , as a marker of vascular remodelling) [23] , F4/80 (as a marker of macrophages) [24] , [25] and IL-6 (as a marker of inflammation) [16] , [26] , [27] , [28] , [29] , [30] were seen in the aorta ( Fig. 1f ). 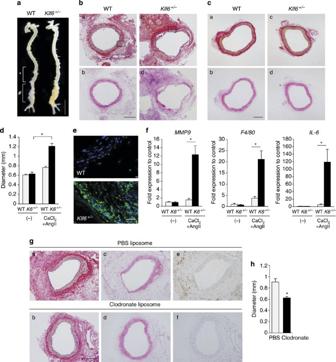Figure 1: Aortic aneurysm and inflammation inKlf6heterozygous knockout mice. (a) Representative aorta (infrarenal aorta: hash, suprarenal aorta: asterisk) induced by 2 weeks of AngII infusion with CaCl2application in wild-type (WT) littermates (n=11) andKlf6heterozygous knockout (Klf6+/−,n=10) mice. Scale bar, 5 mm. Histopathological analysis of infrarenal (b) and suprarenal aorta (c) by EVG (upper panels, a and c) and haematoxylin/eosin (H&E) staining (lower panels, b and d). Scale bar, 200 μm. (d) Quantification of infrarenal aortic diameters between WT littermates andKlf6heterozygous knockout (K6+/−) mice before ((−),n=3) and after 2 weeks of AngII infusion with CaCl2application (CaCl2+AngII, WT;n=10,K6+/−;n=8). *P<0.05, Student’st-test. (e) Immunofluorescent staining for macrophages (green: Mac3, blue: DAPI) in boxed area of EVG-stained aorta (b) of WT littermates andKlf6heterozygous knockout mice. Scale bar, 30 μm. (f) Expression of RNA levels ofMMP9,F4/80andIL-6in aorta from WT littermates andKlf6heterozygous knockout (K6+/−) mice before ((−),n=3) and after AngII infusion with CaCl2application (CaCl2+AngII,n=5) as examined using real-time PCR and normalized byGAPDHmessenger RNA. *P<0.05, Mann–Whitney test. (g) Inhibitory effect of clodronate liposomes on aortic phenotype (n=4) compared with PBS-liposome-administered mice (n=5) by EVG (left panels, a and b); H&E (middle panels, c and d); and F4/80 staining (right panels, e and f, immunohistochemistry). Scale bar, 200 μm. (h) Quantification of infrarenal aortic diameters from clodronate-liposome- or PBS-liposome-administered mice (*P<0.05, Student’st-test,n=4 or 5 mice per group). Results are from three independent experiments. All values are presented as means±s.e.m. Figure 1: Aortic aneurysm and inflammation in Klf6 heterozygous knockout mice. ( a ) Representative aorta (infrarenal aorta: hash, suprarenal aorta: asterisk) induced by 2 weeks of AngII infusion with CaCl 2 application in wild-type (WT) littermates ( n =11) and Klf6 heterozygous knockout ( Klf6 +/− , n =10) mice. Scale bar, 5 mm. Histopathological analysis of infrarenal ( b ) and suprarenal aorta ( c ) by EVG (upper panels, a and c) and haematoxylin/eosin (H&E) staining (lower panels, b and d). Scale bar, 200 μm. ( d ) Quantification of infrarenal aortic diameters between WT littermates and Klf6 heterozygous knockout ( K6 +/− ) mice before ((−), n =3) and after 2 weeks of AngII infusion with CaCl 2 application (CaCl 2 +AngII, WT; n =10, K6 +/− ; n =8). * P <0.05, Student’s t -test. ( e ) Immunofluorescent staining for macrophages (green: Mac3, blue: DAPI) in boxed area of EVG-stained aorta ( b ) of WT littermates and Klf6 heterozygous knockout mice. Scale bar, 30 μm. ( f ) Expression of RNA levels of MMP9 , F4/80 and IL-6 in aorta from WT littermates and Klf6 heterozygous knockout ( K6 +/− ) mice before ((−), n =3) and after AngII infusion with CaCl 2 application (CaCl 2 +AngII, n =5) as examined using real-time PCR and normalized by GAPDH messenger RNA. * P <0.05, Mann–Whitney test. ( g ) Inhibitory effect of clodronate liposomes on aortic phenotype ( n =4) compared with PBS-liposome-administered mice ( n =5) by EVG (left panels, a and b); H&E (middle panels, c and d); and F4/80 staining (right panels, e and f, immunohistochemistry). Scale bar, 200 μm. ( h ) Quantification of infrarenal aortic diameters from clodronate-liposome- or PBS-liposome-administered mice (* P <0.05, Student’s t -test, n =4 or 5 mice per group). Results are from three independent experiments. All values are presented as means±s.e.m. Full size image As marked infiltration of immune cells was seen in the diseased aorta of these mice, macrophages were depleted using clodronate, which abrogated the aortic phenotype with near absence of macrophage infiltration ( Fig. 1g,h ). Thus, immune cells including macrophages were important for aortic remodelling in this model. Klf6 fl/fl ;LysM Cre mice exhibit aortic dissection/haematoma As the aortic condition in Klf6 -deficient mice appeared to involve a dysregulated inflammatory response by macrophages, myeloid-specific Klf6 -deficient mice ( Klf6 fl/fl ;LysM Cre mice) were further generated, which showed specific reduction of KLF6 expression in the myeloid lineage by 70% as compared with control mice. Klf6 fl/fl ;LysM Cre mice subjected to aortic inflammation showed a similar phenotype of exacerbated abdominal aortic aneurysm to that seen in heterozygous knockout mice ( Fig. 2a,b ), but intriguingly, further showed suprarenal aortic dissection/intramural haematoma defined as separation of the intra-aortic wall with haematoma formation accompanied by intimal tear for dissection [3] ( Fig. 2c–f ). Mice that died were from aortic rupture most likely secondary to aortic dissection/intramural haematoma ( Fig. 2g ). This lesion also showed fibrotic tissue deposition with infiltration of Mac3-positive macrophages ( Fig. 3a,b ), thus confirming that the aortic phenotype in KLF6 deficiency was associated with perturbation of the inflammatory response. 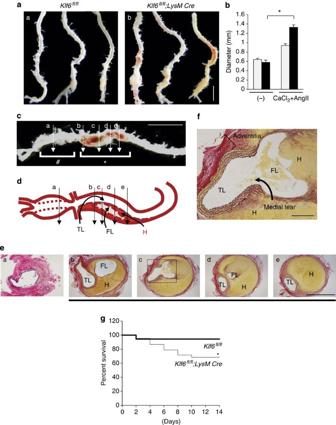Figure 2: MyeloidKlf6-deficient mice show aortic dissection/haematoma. (a) Representative aorta ofKlf6fl/flcontrol mice (a) andKlf6fl/fl;LysM Cremice (b) after 2 weeks of AngII infusion with CaCl2application. Scale bar, 5 mm. (b) Quantification of infrarenal aortic diameters before ((−),n=3) and after 2 weeks of AngII infusion with CaCl2application (CaCl2+AngII,n=5). Results are from three independent experiments. All values are presented as means±s.e.m. *P<0.05, Student’st-test. (c) Thoracic-abdominal aorta subjected to CaCl2application and AngII infusion (infrarenal aorta: hash, suprarenal aorta: asterisk). Note that intramural thrombus formation is present in the suprarenal region. Scale bar, 5 mm. (d) Schematic illustration of the diseased aorta (TL: true lumen, FL: false lumen, H: haematoma). (e) Cross-sectional histological sections stained by Elastica van Gieson. (a) Cross-section of the infrarenal abdominal aorta (CaCl2application region). (b) At the level of the renal arteries. (c) Suprarenal level where the intima-medial layer shows a tear. (d and e) Suprarenal descending thoracic aorta beyond the intima-medial tear. Scale bar, 1 mm. (f) High-magnification cross-section at the suprarenal level (e(c, boxed)). Intima-medial tear and false lumen/mural thrombus formation are present. Scale bar, 200 μm. (g) Survival curve betweenKlf6fl/flcontrol mice (n=19) andKlf6fl/fl;LysM Cremice (n=22) with CaCl2application and AngII infusion. *P<0.05, log-rank test. Figure 2: Myeloid Klf6 -deficient mice show aortic dissection/haematoma. ( a ) Representative aorta of Klf6 fl/fl control mice ( a ) and Klf6 fl/fl ;LysM Cre mice ( b ) after 2 weeks of AngII infusion with CaCl 2 application. Scale bar, 5 mm. ( b ) Quantification of infrarenal aortic diameters before ((−), n =3) and after 2 weeks of AngII infusion with CaCl 2 application (CaCl 2 +AngII, n =5). Results are from three independent experiments. All values are presented as means±s.e.m. * P <0.05, Student’s t -test. ( c ) Thoracic-abdominal aorta subjected to CaCl 2 application and AngII infusion (infrarenal aorta: hash, suprarenal aorta: asterisk). Note that intramural thrombus formation is present in the suprarenal region. Scale bar, 5 mm. ( d ) Schematic illustration of the diseased aorta (TL: true lumen, FL: false lumen, H: haematoma). ( e ) Cross-sectional histological sections stained by Elastica van Gieson. (a) Cross-section of the infrarenal abdominal aorta (CaCl 2 application region). (b) At the level of the renal arteries. (c) Suprarenal level where the intima-medial layer shows a tear. (d and e) Suprarenal descending thoracic aorta beyond the intima-medial tear. Scale bar, 1 mm. ( f ) High-magnification cross-section at the suprarenal level ( e (c, boxed)). Intima-medial tear and false lumen/mural thrombus formation are present. Scale bar, 200 μm. ( g ) Survival curve between Klf6 fl/fl control mice ( n =19) and Klf6 fl/fl ;LysM Cre mice ( n =22) with CaCl 2 application and AngII infusion. * P <0.05, log-rank test. 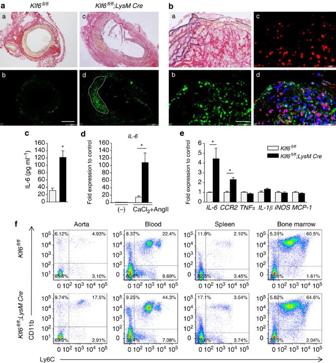Figure 3: Marked inflammation in the aortic lesion of myeloidKlf6-deficient mice. (a) Infiltrated macrophages were visualized by immunofluorescent staining (dotted line, green, Mac3) in aorta ofKlf6fl/fl;LysM Cremice (right panels, c and d) compared withKlf6fl/flmice (left panels, a and b). Scale bar, 100 μm. (b) Immunofluorescent staining for macrophages (b: green, Mac3), pSTAT3 (c: red) and nuclei (d: 4′, 6-diamidino-2-phenylindole, blue) in diseased aorta (a) ofKlf6fl/fl;LysM Cremice. Scale bar, 20 μm. (c) Plasma concentration of IL-6 inKlf6fl/flmice (n=7) andKlf6fl/fl;LysM Cremice (n=9) after 2 weeks of AngII infusion with CaCl2application. *P<0.05, Student’st-test. (d) Expression of RNA levels ofIL-6were examined in aorta fromKlf6fl/flmice andKlf6fl/fl;LysM Cremice before ((−),n=3) and after 2 weeks of AngII infusion with CaCl2application (CaCl2+AngII,n=5) using real-time PCR and normalized byGAPDHmessenger RNA. (e) Expression of RNA levels ofIL-6,CCR2,TNFα,IL-1β,iNOSandMCP-1were examined in bone-marrow-derived macrophages subjected to AngII stimulation (10 μM) for 3 h (n=3 mice per group). (f) Population of CD11b+Ly6Chicells in aorta, peripheral blood, spleen and bone marrow inKlf6fl/flandKlf6fl/fl;LysM Cremice after 2 weeks of AngII infusion with CaCl2application. Results represent three independent experiments. All values are presented as means±s.e.m. *P<0.05, Mann–Whitney test (d,e). Full size image Figure 3: Marked inflammation in the aortic lesion of myeloid Klf6 -deficient mice. ( a ) Infiltrated macrophages were visualized by immunofluorescent staining (dotted line, green, Mac3) in aorta of Klf6 fl/fl ;LysM Cre mice (right panels, c and d) compared with Klf6 fl/fl mice (left panels, a and b). Scale bar, 100 μm. ( b ) Immunofluorescent staining for macrophages (b: green, Mac3), pSTAT3 (c: red) and nuclei (d: 4′, 6-diamidino-2-phenylindole, blue) in diseased aorta (a) of Klf6 fl/fl ;LysM Cre mice. Scale bar, 20 μm. ( c ) Plasma concentration of IL-6 in Klf6 fl/fl mice ( n =7) and Klf6 fl/fl ;LysM Cre mice ( n =9) after 2 weeks of AngII infusion with CaCl 2 application. * P <0.05, Student’s t -test. ( d ) Expression of RNA levels of IL-6 were examined in aorta from Klf6 fl/fl mice and Klf6 fl/fl ;LysM Cre mice before ((−), n =3) and after 2 weeks of AngII infusion with CaCl 2 application (CaCl 2 +AngII, n =5) using real-time PCR and normalized by GAPDH messenger RNA. ( e ) Expression of RNA levels of IL-6 , CCR2 , TNFα , IL-1β , iNOS and MCP-1 were examined in bone-marrow-derived macrophages subjected to AngII stimulation (10 μM) for 3 h ( n =3 mice per group). ( f ) Population of CD11b + Ly6C hi cells in aorta, peripheral blood, spleen and bone marrow in Klf6 fl/fl and Klf6 fl/fl ;LysM Cre mice after 2 weeks of AngII infusion with CaCl 2 application. Results represent three independent experiments. All values are presented as means±s.e.m. * P <0.05, Mann–Whitney test ( d , e ). Full size image Mechanistically, Klf6 fl/fl ;LysM Cre mice showed elevated expression of IL-6 in the aortic lesion ( Fig. 3d ) and elevated circulating levels ( Fig. 3c ). Further, macrophages obtained from bone marrow of Klf6 fl/fl ;LysM Cre mice exhibited increased IL-6 expression ( Fig. 3e ). Differences in expression were not seen in other major pro-inflammatory cytokines such as IL-1β , MCP-1 or TNFα between macrophages from Klf6 fl/fl and Klf6 fl/fl ;LysM mice ( Fig. 3e ). Immune cells in the diseased aorta of these mice were characterized by flow cytometry analysis, which showed a markedly increased population of CD11b + Ly6C hi inflammatory monocytes and this increase was also seen in the peripheral blood ( Fig. 3f ). Granulocytes (for example, neutrophils; Ly6G + cells) were not affected in number or (sub)population under basal conditions or in the setting of CaCl 2 and AngII infusion ( Supplementary Table 1 ; Supplementary Fig. 1a,c ), nor was the functional activity of neutrophils, as examined by inflammatory cytokine expression such as IL-8 or TNFα [31] ( Supplementary Fig. 1e ), or that of the population of dendritic cells (Lineage − CD11c + cells) ( Supplementary Fig. 1b,d ) affected under these conditions. Taken together, expansion of inflammatory monocytes in the aorta and circulation was selectively associated with the present experimental model and conditions. TGFβ, a central molecule in the pathogenesis of Marfan aortopathy [12] , [14] , [32] , [33] , [34] , and its downstream signalling pathways (canonical pSmad2 (ref. 35 ) and non-canonical pERK1/2 (ref. 12 )) were not affected in either Klf6 fl/fl ;LysM Cre mice or heterozygous knockout mice, while pSTAT3, a downstream signalling pathway of IL-6, was activated in both mice ( Fig. 4a–d ), suggesting that the TGFβ-mediated pathway was not critically involved in the underlying phenotype, and that the IL-6/STAT3 pathway is. 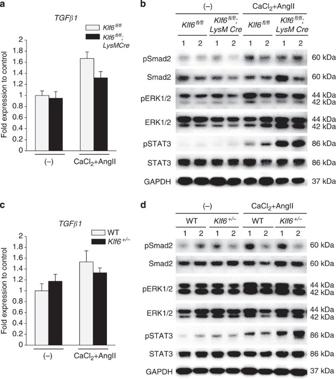Figure 4: Involvement of TGFβ pathways in aortic dissection/haematoma. Expression of messenger RNA (mRNA) levels of TGFβ1-related factors in aorta fromKlf6fl/flandKlf6fl/fl;LysM Cremice (a), and in wild-type (WT) littermates andKlf6+/−mice (c), using real-time PCR normalized byGAPDHmRNA.n=5 per group. All values are presented as mean±s.e.m. Western blot analysis for pSmad2, Smad2, pERK1/2, ERK1/2, pSTAT3, STAT3 or GAPDH in aorta before (−) and after 2 weeks of AngII infusion with CaCl2application (CaCl2+AngII) inKlf6fl/flandKlf6fl/fl;LysM Cremice (b) and WT littermates andKlf6+/−mice (d). Results represent three independent experiments. Figure 4: Involvement of TGFβ pathways in aortic dissection/haematoma. Expression of messenger RNA (mRNA) levels of TGFβ1-related factors in aorta from Klf6 fl/fl and Klf6 fl/fl ;LysM Cre mice ( a ), and in wild-type (WT) littermates and Klf6 +/− mice ( c ), using real-time PCR normalized by GAPDH mRNA. n =5 per group. All values are presented as mean±s.e.m. Western blot analysis for pSmad2, Smad2, pERK1/2, ERK1/2, pSTAT3, STAT3 or GAPDH in aorta before (−) and after 2 weeks of AngII infusion with CaCl 2 application (CaCl 2 +AngII) in Klf6 fl/fl and Klf6 fl/fl ;LysM Cre mice ( b ) and WT littermates and Klf6 +/− mice ( d ). Results represent three independent experiments. Full size image GM-CSF is a downstream target of KLF6 Delineation of target molecules and mechanisms of regulation of immune cells was next addressed using RNA profiling array analysis. Remarkably, GM-CSF levels showed the greatest increase in macrophages derived from bone marrow of Klf6 fl/fl ;LysM Cre mice in response to AngII stimulation (3.89-fold) as compared with control macrophages ( Fig. 5a ). Macrophages obtained from the aorta of Klf6 fl/fl ;LysM Cre mice showed markedly increased expression of GM-CSF under experimental conditions of CaCl 2 application and AngII infusion ( Fig. 5b ), and in macrophages derived from bone marrow of these mice ( Supplementary Fig. 2a ). Expression of GM-CSF in the aorta was elevated from 3 days after treatment (before onset of aortic dissection) of Klf6 fl/fl ;LysM Cre mice ( Fig. 5c ). Whether deletion of KLF6 in macrophages affects secretion of GM-CSF and further systemic circulating levels was next asked. Macrophages and GM-CSF co-localized in the aorta of Klf6 fl/fl ;LysM Cre mice, and GM-CSF was markedly produced by macrophages in response to pro-inflammatory stimuli ( Fig. 5d ; Supplementary Fig. 2b ). Circulating levels of GM-CSF were at least 73.3-fold higher in Klf6 -deleted mice ( Fig. 5e ). It therefore seems that a markedly increased response in GM-CSF is a hallmark feature of the aorta in Klf6 fl/fl ;LysM Cre mice. 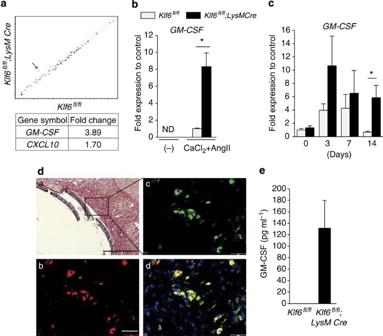Figure 5: GM-CSF is a direct target of KLF6 in macrophages. (a) RT2 profiler PCR array analysis of genes related to IL-6/STAT3 inflammatory pathway between bone marrow (BM)-derived macrophages fromKlf6fl/flandKlf6fl/fl;LysM Cremice with AngII stimulation (10 μM) for 3 h. Arrow indicatesGM-CSF. List of genes that showed consistent changes between BM-derived macrophages fromKlf6fl/flandKlf6fl/fl;LysM Cremice stimulated with AngII (10 μM) for 3 h. (b) Messenger RNA (mRNA) expression ofGM-CSFin aortic macrophages obtained fromKlf6fl/fl(sham; (−),n=3; CaCl2+AngII;n=3) andKlf6fl/fl;LysM Cremice (sham; (−),n=3; CaCl2+AngII;n=6). ND indicates not detected. (c) mRNA expression ofGM-CSFin aorta ofKlf6fl/flandKlf6fl/fl;LysM Cremice at 0 (n=3), 3 (n=3), 7 (n=3) and 14 (n=4) days. (d) Immunohistochemistry for macrophages (red: F4/80, b; scale bar, 30 μm), GM-CSF (green: c) and nucleus (blue: 4′, 6-diamidino-2-phenylindole, d) in aorta ofKlf6fl/fl;LysM Cremice with EVG-stained infrarenal aorta (a, scale bar, 200 μm). (e) Plasma GM-CSF concentration betweenKlf6fl/fl(n=8) andKlf6fl/fl;LysM Cremice (n=4) after 2 weeks of AngII infusion with CaCl2application. Results represent three independent experiments. All values are presented as means±s.e.m. *P<0.05, Mann–Whitney test. Figure 5: GM-CSF is a direct target of KLF6 in macrophages. ( a ) RT2 profiler PCR array analysis of genes related to IL-6/STAT3 inflammatory pathway between bone marrow (BM)-derived macrophages from Klf6 fl/fl and Klf6 fl/fl ;LysM Cre mice with AngII stimulation (10 μM) for 3 h. Arrow indicates GM-CSF . List of genes that showed consistent changes between BM-derived macrophages from Klf6 fl/fl and Klf6 fl/fl ;LysM Cre mice stimulated with AngII (10 μM) for 3 h. ( b ) Messenger RNA (mRNA) expression of GM-CSF in aortic macrophages obtained from Klf6 fl/fl (sham; (−), n =3; CaCl 2 +AngII; n =3) and Klf6 fl/fl ;LysM Cre mice (sham; (−), n =3; CaCl 2 +AngII; n =6). ND indicates not detected. ( c ) mRNA expression of GM-CSF in aorta of Klf6 fl/fl and Klf6 fl/fl ;LysM Cre mice at 0 ( n =3), 3 ( n =3), 7 ( n =3) and 14 ( n =4) days. ( d ) Immunohistochemistry for macrophages (red: F4/80, b; scale bar, 30 μm), GM-CSF (green: c) and nucleus (blue: 4′, 6-diamidino-2-phenylindole, d) in aorta of Klf6 fl/fl ;LysM Cre mice with EVG-stained infrarenal aorta (a, scale bar, 200 μm). ( e ) Plasma GM-CSF concentration between Klf6 fl/fl ( n =8) and Klf6 fl/fl ;LysM Cre mice ( n =4) after 2 weeks of AngII infusion with CaCl 2 application. Results represent three independent experiments. All values are presented as means±s.e.m. * P <0.05, Mann–Whitney test. Full size image We next sought to understand mechanisms underlying regulation of GM-CSF expression and secretion by KLF6. Overexpression of KLF6 significantly attenuated GM-CSF expression induced by pro-inflammatory stimuli in macrophages ( Supplementary Fig. 2c ). Transcriptionally, several KLF-binding sites were present in the promoter region of GM-CSF to which KLF6 was recruited by agonistic stimuli treatment in macrophages ( Supplementary Fig. 2d ). These results demonstrated that, mechanistically, GM-CSF is a direct target of KLF6 and that KLF6 represses expression of GM-CSF. GM-CSF manipulation regulates aortic dissection/haematoma To next test the requirement of GM-CSF in aortic dissection in these mice, the actions of GM-CSF were blocked using a neutralizing antibody, which abrogated aortic dissection/intramural haematoma ( Fig. 6a,b ) as well as expression of GM-CSF receptor α, MMP9 , F4/80 and IL-6 ( Fig. 6d ) in addition to serum levels of IL-6 ( Fig. 6c ). GM-CSF was therefore required for the aortic phenotype in Klf6 fl/fl ;LysM Cre mice. 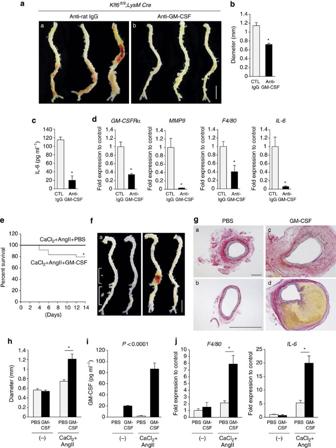Figure 6: GM-CSF is required for aortic dissection/intramural haematoma. (a) Representative aortas ofKlf6fl/fl;LysM Cremice with administration of anti-GM-CSF neutralizing antibody (b, anti-GM-CSF,n=8) or control IgG antibody (a,n=10) after 2 weeks of AngII infusion with CaCl2application. Scale bar, 5 mm. Quantification of infrarenal aortic diameters (b, anti-GM-SCF:n=7; anti-control IgG:n=9) and plasma concentration of IL-6 (c,n=5 or 6) between anti-GM-CSF antibody-administered and anti-control IgG-administered mice. *P<0.05, Student’st-test. (d) Expression levels of RNA ofGM-CSFRα,MMP9,F4/80andIL-6were examined in aorta of anti-GM-CSF antibody-administered mice or anti-control IgG-administered mice using real-time PCR and then normalized byGAPDHmessenger RNA (mRNA) (n=5 mice per group). (e) Survival curve of mice with administration of recombinant GM-CSF (n=26) or PBS (n=19) with CaCl2application and AngII infusion in wild-type mice. *P<0.05, log-rank test. (f) Representative aorta of wild-type mice with administration of recombinant GM-CSF (b) or PBS (a) with CaCl2application and AngII infusion (infrarenal aorta: hash, suprarenal aorta: asterisk) for 4 weeks. Scale bar, 5 mm. (g) Histopathological analysis of infrarenal aorta (upper panels: a and c, scale bar, 200 μm) and suprarenal aorta (lower panels: b and d, scale bar, 1 mm) by EVG staining. (h) Quantification of infrarenal aortic diameters between recombinant GM-CSF-administered mice or PBS-administered mice (sham; (−),n=3, CaCl2+AngII;n=5). (i) Plasma GM-CSF concentration after 2 weeks infusion of recombinant GM-CSF or PBS with or without CaCl2application and AngII infusion (n=3∼5 mice per group). (j) Expression levels of RNA ofF4/80andIL-6were examined in aorta from mice administered recombinant GM-CSF or PBS using real-time PCR and then normalized withGAPDHmRNA (sham; (−),n=3, CaCl2+AngII;n=5). Results are from three independent experiments. All values are presented as means±s.e.m. *P<0.05, Mann–Whitney test (d,h,j) and one-way analysis of variance with Dunn’s post-test (i). Figure 6: GM-CSF is required for aortic dissection/intramural haematoma. ( a ) Representative aortas of Klf6 fl/fl ;LysM Cre mice with administration of anti-GM-CSF neutralizing antibody (b, anti-GM-CSF, n =8) or control IgG antibody (a, n =10) after 2 weeks of AngII infusion with CaCl 2 application. Scale bar, 5 mm. Quantification of infrarenal aortic diameters ( b , anti-GM-SCF: n =7; anti-control IgG: n =9) and plasma concentration of IL-6 ( c , n =5 or 6) between anti-GM-CSF antibody-administered and anti-control IgG-administered mice. * P <0.05, Student’s t -test. ( d ) Expression levels of RNA of GM-CSFRα , MMP9 , F4/80 and IL-6 were examined in aorta of anti-GM-CSF antibody-administered mice or anti-control IgG-administered mice using real-time PCR and then normalized by GAPDH messenger RNA (mRNA) ( n =5 mice per group). ( e ) Survival curve of mice with administration of recombinant GM-CSF ( n =26) or PBS ( n =19) with CaCl 2 application and AngII infusion in wild-type mice. * P <0.05, log-rank test. ( f ) Representative aorta of wild-type mice with administration of recombinant GM-CSF ( b ) or PBS ( a ) with CaCl 2 application and AngII infusion (infrarenal aorta: hash, suprarenal aorta: asterisk) for 4 weeks. Scale bar, 5 mm. ( g ) Histopathological analysis of infrarenal aorta (upper panels: a and c, scale bar, 200 μm) and suprarenal aorta (lower panels: b and d, scale bar, 1 mm) by EVG staining. ( h ) Quantification of infrarenal aortic diameters between recombinant GM-CSF-administered mice or PBS-administered mice (sham; (−), n =3, CaCl 2 +AngII; n =5). ( i ) Plasma GM-CSF concentration after 2 weeks infusion of recombinant GM-CSF or PBS with or without CaCl 2 application and AngII infusion ( n =3 ∼ 5 mice per group). ( j ) Expression levels of RNA of F4/80 and IL-6 were examined in aorta from mice administered recombinant GM-CSF or PBS using real-time PCR and then normalized with GAPDH mRNA (sham; (−), n =3, CaCl 2 +AngII; n =5). Results are from three independent experiments. All values are presented as means±s.e.m. * P <0.05, Mann–Whitney test ( d , h , j ) and one-way analysis of variance with Dunn’s post-test ( i ). Full size image We further investigated whether GM-CSF is sufficient to induce aortopathy. Administration of GM-CSF in wild-type mice subjected to aortic inflammation (CaCl 2 +AngII) caused aortic dissection/intramural haematoma, confirming the generality of the role of GM-CSF in the pathogenesis of the condition. Mice died from aortic rupture due to the aortic lesion and showed pathological features of the condition (for example, fragile aorta, intimal tear with haematoma) ( Fig. 6e–h,j ). However, aortic dissection/intramural haematoma did not develop by administration of GM-CSF alone, even with abnormally increased circulating levels (at least 180.9-fold) of GM-CSF ( Supplementary Fig. 3a,b ). As AngII, CaCl 2 or GM-CSF alone was not sufficient to induce the condition, it seems that a combination of aortic inflammation with GM-CSF infusion is necessary for the phenotype ( Supplementary Fig. 4a,b ). Consistent with this, circulating levels of GM-CSF in mice were only markedly elevated when treated with the combination of measures as compared with each alone ( Fig. 6i ). Note that these elevated levels were comparable to those in Klf6 fl/fl ;LysM Cre mice, suggesting that highly elevated levels of GM-CSF are required but not sufficient to cause aortic dissection/intramural haematoma ( Fig. 5e ). Finally, whether manipulation of GM-CSF affects the number of peripheral leukocytes was examined. With GM-CSF administration, the number of circulating lymphocytes did not change in either the early phase (5 days) or developed phase (14 days) of the model ( Supplementary Tables 2 and 3 ). With respect to neutrophils, the number in peripheral blood was markedly increased in the early phase, but no difference was observed at 14 days of GM-CSF administration. This was similarly seen in the group in which GM-CSF alone was administered, which did not result in the aortic phenotype. While these changes might be due to acute effects by exogenous GM-CSF treatment, this alone had no bearing on the phenotype. Moreover, the number of circulating granulocytes and lymphocytes was not affected when GM-CSF was depleted by the neutralizing antibody ( Supplementary Table 4 ). On the basis of these results, manipulation of GM-CSF did not affect the number of circulating leukocytes in the present model, at least during the observation period (14 days). Upregulation of GM-CSF in patients with aortic dissection To confirm the clinical relevance of our findings, circulating levels of GM-CSF were measured in sera of patients with acute aortic dissection, which showed marked increases, in contrast to patients with coronary artery disease, aortic aneurysm or healthy volunteers, which showed markedly lower if not negligible levels ( Fig. 7a ). Furthermore, inflammatory infiltration (CD68 + monocytes/macrophage) and GM-CSF expression were upregulated and co-localized in dissected aorta ( Fig. 7b ). Thus, GM-CSF is associated with aortic acute dissection not only in mice but also in human conditions. 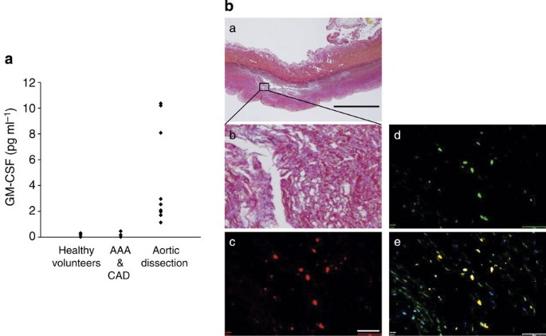Figure 7: Increased GM-CSF in patients with acute aortic dissection. (a) Plasma GM-CSF concentration in healthy volunteers (n=12) and patients with aortic aneurysm (AAA,n=3), coronary artery disease (CAD,n=11) or aortic dissection (n=10). (b) Immunofluorescent staining for CD68 (red, c, scale bar, 50 μm), GM-CSF (green, d) and 4′,6-diamidino-2-phenylindole (blue, e) in descending dissected aorta (boxed area, a, scale bar, 2 mm) with EVG staining (b). Results represent three independent experiments. Figure 7: Increased GM-CSF in patients with acute aortic dissection. ( a ) Plasma GM-CSF concentration in healthy volunteers ( n =12) and patients with aortic aneurysm (AAA, n =3), coronary artery disease (CAD, n =11) or aortic dissection ( n =10). ( b ) Immunofluorescent staining for CD68 (red, c, scale bar, 50 μm), GM-CSF (green, d) and 4′,6-diamidino-2-phenylindole (blue, e) in descending dissected aorta (boxed area, a, scale bar, 2 mm) with EVG staining (b). Results represent three independent experiments. Full size image The present findings show that GM-CSF is a key regulatory molecule causative of aortic dissection/intramural haematoma in a murine model of the condition and to also be associated with the condition in humans. In mice, modulation of GM-CSF by a neutralizing antibody or exogenous administration, respectively, prevented or induced onset of this phenotype. In humans, elevated serum GM-CSF levels and expression of the cytokine in aortic tissue were seen in patients with aortic dissection. GM-CSF was a central component of the aortic dissection/intramural haematoma phenotype in our murine model. Previous studies had suggested a limited role of GM-CSF in the pathogenesis of aortic disease [36] , [37] , [38] , [39] . For example, mice that lack Smad3 manifested a phenotype of aortic aneurysm formation [39] , and GM-CSF was shown to play a pivotal role in the pathogenesis; however, it was assumed that because smad3 is a downstream target of TGFβ, which is a central molecule associated in Marfan aortopathy, the pathogenic mechanism was limited to this genetic aortopathy. Our findings show that activation of the GM-CSF pathway in a manner independent of the TGFβ-SMAD pathway is sufficient to trigger this condition in a model of inflammatory and degenerative aorta (calcium chloride treatment causes stiffening of the aorta to mimic the condition as seen in atherosclerotic human aortas [40] ). This model is reflective of aortic dissection/intramural haematoma seen in the elderly adult in humans and should be differentiated from the genetic aortopathy in young patients with Marfan syndrome.. GM-CSF tissue expression had also been shown to be increased in a patient presenting with aortic dissection in Cogan’s disease [41] , an apparently autoimmune condition that is characterized by recurrent corneal inflammation [42] , which was thought to be an isolated finding. Effects on other non-macrophage myeloid cells were investigated, which showed that dendritic cells (CD11c + MHCII + cells) were increased in the diseased aorta but not in the circulation under KLF6-deficient conditions, and lack of effects on neutrophils (Ly6G + cells) either in the circulation or in the aortic tissue ( Supplementary Fig. 1 ; Supplementary Fig. 5 ). The contributory role of non-macrophage myeloid cells (for example, dendritic cells) needs to be further investigated. Macrophage colony-stimulating factor (M-CSF) has been also suggested to be an important regulator of vascular remodelling [43] , [44] . Although the precise molecular mechanisms of the actions of M-CSF are still unclear, different actions as compared with GM-CSF are envisioned, given different expression patterns in the vascular wall. Whereas M-CSF is constitutively expressed under physiological conditions in endothelial cells, fibroblasts, macrophages and smooth muscle cells, GM-CSF, by contrast, is expressed only in minute amounts in these cells under basal conditions, but instead is induced by inflammatory stimuli (for example, tumour necrosis factor) [45] or oxidized low-density lipoprotein cholesterol stimulation [46] . In murine and human lesions, M-CSF is detected both in healthy arteries and in atherosclerotic lesions associated with macrophage and foam cell content, and is correlated with plaque progression in the latter. By contrast, only minute levels of GM-CSF are seen in smooth muscle cells and endothelial cells of healthy human arteries, but are elevated upon atherosclerotic development and macrophage accumulation [47] . On the basis of these observations, collectively, while M-CSF is a constitutively expressed cytokine in the vasculature, GM-CSF is markedly induced in diseased vessels to regulate pathological conditions including the described aortopathy. In the experimental model, most previous studies have used AngII infusion alone as an intervention to induce a dissection phenotype [16] , [48] . However, the limitation of this procedure for mechanistic investigations including inflammation was the low reproducibility (less than 30%), need for long-term infusion of AngII (more than 4 weeks) and incidence/expression of phenotype in aged mice (over 7–10 months age) with a specific genetic background ( apoE −/− or ldl receptor −/− mice). Most noteworthy is that the present model could induce aortic dissection/intramural haematoma within 2 weeks with high reproducibility (at least 70%) even in young wild-type mice. Mechanistically, this model might involve hemodynamic stress on the suprarenal dissection site due to loss of Windkessel effect [49] because of increased stiffening in the infrarenal aorta (for example, downward shift of the pressure-diameter curve after CaCl 2 application with continuous AngII infusion) [40] that showed aneurysmal formation, which when exposed to inflammatory effects of GM-CSF triggered dissection/intramural haematoma formation in the weak and fragile suprarenal aorta. As aortic aneurysm is commonly co-present in patients with dissection [4] , the described animal model and findings closely resemble the condition seen in patients. Taken together, our findings suggest that GM-CSF is a central regulator of aortic dissection/intramural haematoma in the atherosclerotic and inflammatory aorta, which is typically seen in the elderly patient with this condition, and may serve as a potential target for diagnostic and therapeutic exploitation (for example, aortic stabilization using GM-CSF antagonists), as well as a diagnostic biomarker. Mice Heterozygous Klf6 +/− mice (C57BL/6) were originally generated by Tarocchi et al. [50] To generate macrophage-specific Klf6 -knockout mice, Klf6 fl/fl mice (C57BL/6;129Sv) were cross-bred with LysM Cre mice (C57BL/6, Jackson laboratory) [51] . Only male mice, 10- to 13-weeks of age, and C57BL/6 as wild-type mouse (CLEA Japan) were used. All experimental protocols were approved by the Ethics Committee for Animal Experimentation at the Graduate School of Medicine, the University of Tokyo, and conducted in accordance with the Guidelines for the Care and Use of Laboratory Animals of the Department of Medicine, the University of Tokyo. Murine aortic dissection/intramural haematoma model To induce aortic dissection/intramural haematoma, peri-aortic application of CaCl 2 was performed on the abdominal aorta, followed by a 2-week infusion of AngII (2,000 ng kg −1 min −1 ) [40] . In detail, mice were anaesthetized and underwent laparotomy at 10–13 weeks of age. The abdominal aorta between the renal arteries and bifurcation of the iliac arteries was isolated from the surrounding retroperitoneal structure, and 0.5 M CaCl 2 was applied to the external surface of the infrarenal aorta. NaCl (0.9%) was substituted for CaCl 2 in sham control mice. The aorta was rinsed with 0.9% sterile saline after 15 min and the incision was closed. Macrophage depletion and manipulation of GM-CSF Wild-type mice were injected intraperitoneally with 110 mg kg −1 of clodronate liposomes or equal volume of PBS liposomes 2 days prior and 7 days after induction of aortic dissection. Neutralizing antibody against GM-CSF (300 μg, R&D systems) or control anti-rat IgG antibody (Equitech Bio) was administered every other day by intraperitoneal injection. Recombinant murine GM-CSF (10, 50 and 100 μg kg −1 per day, PeproTech) was administered for 2 or 4 weeks after induction of aortic dissection. Histological analysis and immunohistochemistry Aortas from mice were embedded in paraffin and then 5-μm-thick serial sections were prepared for Elastic Van Gienson (EVG) and haematoxylin/eosin staining. Digital images of EVG-stained aortas with a reference scale were used for absolute measurement of diameter. Human aortic tissue was obtained from patients undergoing surgical aortic repair with informed consent under a protocol approved by the University of Tokyo Hospital Research Ethics Committee. Paraffin-embedded sections were taken from the aorta for EVG staining and immunohistochemistry. For immunohistochemistry, after deparaffinization and blocking, serial sections were incubated with the following antibodies: Mac3 (dilution 1:200; rat; BD Pharmingen) or F4/80 (1:100; rat; Serotec) for macrophages in mice and CD68 (1:50; mouse; Dako) in humans and GM-CSF (1:100, rabbit; Abcam for mouse and 1:50; rabbit; Acris for humans) or pSTAT3 (1:200; rabbit; Cell Signaling Technology), followed by biotinylated secondary antibodies (1:200; Dako). For detection, anti-streptavidin-conjugated AlexFluor 488 or AlexFluor 594 (1:200; Invitrogen) was used. The nuclei were stained with 4′, 6-diamidino-2-phenylindole (1:5,000; Sigma-Aldrich) after the final series of washes. Cell preparation from aorta, spleen, bone marrow and blood Aortas were minced into 3- to 4-mm pieces and placed in 1 ml digestion solution containing collagenase type II (1.25 mg ml −1 , Worthington) and porcine pancreatic elastase (50 μg ml −1 , Worthington) in a base solution of Accumax (Innovative Cell Technologies). Aortic tissue was digested at room temperature with agitation for 1 h. After digestion, cells were washed in FACS buffer (5% FCS in PBS) at 2,000 r.p.m. for 5 min (ref. 16 ). Aortic macrophages were isolated using CD11b microbeads according to the manufacturer’s instructions (Miltenyi Biotec). Spleen was homogenized and passed through a cell strainer to obtain single-cell suspensions. Bone-marrow-derived cells were taken from the femur and tibia of 5–6-week-old mice. Blood was collected in heparin-coated vials and then 1.2% dextran was added for 45 min at room temperature. Counting of peripheral leukocytes was done by an automated hematology analyzer (XT-2,000i, Sysmex). Neutrophils were isolated from bone marrow using a neurophil isolation kit according to the manufacturer’s instructions (Miltenyi Biotec). From single-cell suspensions of spleen, bone marrow and blood, erythrocytes were lysed using ACK lysis buffer for 5, 3 and 2 min on ice, respectively. Cells were centrifuged at 2,000 r.p.m. for 5 min to remove the ACK lysis buffer, then the single-cell suspensions were resuspended and washed in FACS buffer, followed by centrifugation at 2,000 r.p.m. for 5 min. Cell cultures Bone-marrow-derived cells were prepared from femur and tibia of Klf6 fl/fl mice or Klf6 fl/fl ;LysM Cre mice to assess the role of GM-CSF in macrophages. KLF6 overexpression was induced by a retrovirus construct for KLF6 (pMXs-KLF6) in the presence of RetroNectin (5 μg cm −2 , Takara Bio.). Flow cytometry Murine Fc receptors were blocked using antibodies against murine CD16/32 antigens (eBioscience) for 15 min on ice, after which cells were washed and then resuspended in 100 μl FACS buffer. Fluorochrome-conjugated antibodies (all from BioLegend) for APC-CD11b[M1/70], PerCP-Cy5.5-Ly-6c[HK1.4], APC-Cy7-Ly6G[1A8] or APC-CD11c[N418] were added for 30–45 min at room temperature. FITC-CD3e[145-2C11], FITC-Ly6G[RB6-8C5], FITC-CD11b[M1/70], FITC-CD45R/B220[RA3-6B2] and FITC-Ly76[Ter-119] (erythroid lineage marker) were used as lineage markers. Corresponding isotype control antibodies were added to samples at the same concentrations as the antibodies of interest. After incubation, samples were washed three times and analysed by FACSverse (BD Pharmingen). Compensation was done using positive samples containing single-colour-stained aortic macrophages. Debris and dead cells, as defined by low forward scatter, were excluded from analysis. Data were analysed with FlowJo (Tree Star) (ref. 16 ). Chromatin immunoprecipitation Chromatin immunoprecipitation analysis was performed using a Chromatin Immunoprecipitation Kit (Active Motif) according to the manufacturer’s instructions. Briefly, bone-marrow-derived macrophages were stimulated with or without AngII (10 μM), TNF α (10 ng ml −1 ) and IL-1β (20 ng ml −1 ) for 3 h prior to crosslinking for 10 min with 1% formaldehyde. Chromatin was sheared by sonication to an average size of 200 ∼ 1,000 base pairs (Covaris). Immunoprecipitation was performed using anti-KLF6 antibody (25 ng μl −1 , Santa Cruz Biotechnology) and rabbit IgG antibody (25 ng μl −1 , Santa Cruz Biotechnology). PCR amplification of the GM-CSF promoter region spanning KLF-binding elements was performed using the following primers: forward: 5′-AAGC CCTTCCAAGAACTGGC-3′ and reverse 5′-GGCCCCTCAAAAAGGAGAGG-3′. KLF6 recruitment was normalized by input DNA and compared with the control group using KLF6 antibody. RNA isolation and quantitative real-time PCR Total RNA from cultured cells, aortic macrophages, bone-marrow-derived neutrophils or murine aortic samples was extracted using either the RNeasy minikit (Qiagen) or RNA later (Qiagen) according to the manufacturer’s instructions. In total, 0.5–1 μg RNA was reverse-transcribed using Superscript III (Invitrogen) according to the manufacturer’s instructions. Real-time PCRs were performed using 2 μl of resulting cDNA per 20-μl reaction volume containing SYBR green I master (Roche). Glyceraldehyde 3-phosphate dehydrogenase was used as an internal control. Using bone-marrow-derived macrophages with AngII (10 μM, 3 h) stimulation, RT2 profiler PCR array (Qiagen) was performed with 84 related genes for the IL-6/STAT inflammatory pathway. PCR was performed on a LightCycler 480 Real-time PCR system (Roche) in accordance with the manufacturer’s recommended procedure. Real-time PCR primers are shown in Supplementary Table 5 . Western blot analysis Mouse aortic specimens were homogenized with lysis buffer (T-PER, Thermo Scientific) containing the protease inhibitor complex (Roche) and phosphatase inhibitors (Roche). Protein concentration was assayed using the BCA protein assay kit (Pierce), and 5 μg of the protein were resolved by 10% NuPAGE (Invitrogen) and then transferred to polyvinylidene difluoride membrane. The blot was probed with primary antibodies: pSmad2 (dilution 1:400), pERK1/2 (1:3,000), pSTAT3 (1:3,000), Smad2 (1:1,000), ERK1/2 (1:3,000) or STAT3 (1:3,000) (all rabbit antibodies obtained from Cell Signaling Technology) and anti-GAPDH antibody (1:1,000, Ambion). Membranes were washed and incubated with the corresponding horseradish peroxidase-conjugated secondary antibody (Cell Signaling Technology). Protein bands were detected by ECLplus (Thermo scientific) and GAPDH served as an internal control for protein loading. The original blots for the representative images are displayed in Supplementary Fig. 6 . Enzyme-linked immunosorbent assay Plasma levels of IL-6, MCP-1 and GM-CSF in mice or in humans with or without aortic dissection/intramural haematoma were assayed with commercially available quantikine ELISA kits (R&D systems) according to the manufacturer’s instructions. Sera of healthy volunteers and of patients with aortic aneurysm, coronary artery disease or with aortic dissection were obtained with informed consent under a protocol approved by the University of Tokyo Hospital Research Ethics Committee. Baseline characteristics of human subjects are shown in Supplementary Table 6 . Statistical analyses All data are presented as means±s.e.m. Statistical difference between two groups was determined using the Student’s t -test (two-tailed) for parametric data or the Mann–Whitney test for non-parametric data after testing for normality by F-test analysis. For data containing multiple time points, two group comparisons at the same time point were done. When comparing multiple groups, data were analysed by the Kruskal–Wallis non-parametric one-way analysis of variance with Dunn’s post-test. Survival curves were created using the Kaplan–Meier method and compared by a log-rank test. Statistical power for mouse experiments was calculated using Biomath (biomath.info/power). All samples sizes were equal to or greater than the recommended minimum group size. All data were analysed using Prism 6.0 (GraphPad Software). A P value of less than 0.05 was considered significant. How to cite this article: Son, B.-K. et al. Granulocyte macrophage colony-stimulating factor is required for aortic dissection/intramural haematoma. Nat. Commun. 6:6994 doi: 10.1038/ncomms7994 (2015).